Combinatorial effects on gene expression at theLbx1/Fgf8locus resolve split-hand/foot malformation type 3 Split-Hand/Foot Malformation type 3 (SHFM3) is a congenital limb malformation associated with tandem duplications at the LBX1 / FGF8 locus. Yet, the disease patho-mechanism remains unsolved. Here we investigate the functional consequences of SHFM3-associated rearrangements on chromatin conformation and gene expression in vivo in transgenic mice. We show that the Lbx1 / Fgf8 locus consists of two separate, but interacting, regulatory domains. Re-engineering of a SHFM3-associated duplication and a newly reported inversion in mice results in restructuring of the chromatin architecture. This leads to ectopic activation of the Lbx1 and Btrc genes in the apical ectodermal ridge (AER) in an Fgf8- like pattern induced by AER-specific enhancers of Fgf8 . We provide evidence that the SHFM3 phenotype is the result of a combinatorial effect on gene misexpression in the developing limb. Our results reveal insights into the molecular mechanism underlying SHFM3 and provide conceptual framework for how genomic rearrangements can cause gene misexpression and disease. At the sub-megabase scale, chromosomes are organized into distinct regions of high interaction called Topologically Associating Domains (TADs) that are separated from each other by boundaries [1] , [2] . TADs are thought to restrict enhancer-promoter contacts thereby defining regulatory domains. Structural variations (SVs), such as deletions, duplications and inversions, can disrupt these functional units and different types of SVs can induce distinct topological changes. For instance, deletions are mainly responsible for TAD fusion, duplications can promote the formation of a new TAD (neo-TAD), while TAD shuffling is frequently observed upon an inversion [3] , [4] , [5] . SVs can not only affect gene dosage but also modulate basic mechanisms of gene regulation. Indeed, SVs can alter the copy number of regulatory elements or modify the 3D genome by disrupting higher-order chromatin organisation. This can give rise to ectopic enhancer-promoter contacts, gene misregulation and ultimately disease [3] , [4] , [5] , [6] . However, the general applicability of this concept remains under investigation, as disruption of TADs and enhancer-promoter interactions are not always accompanied by changes in expression. Studies in Drosophila [7] and in human congenital chromothrypsis cases [8] indicate indeed a degree of robustness of the genome against such events. SHFM is a congenital limb malformation characterized by variable defects of the central rays of the autopod often together with syndactyly and/or aplasia/hypoplasia of the phalanges, metacarpals, and metatarsals [9] . SHFM is known as a paradigm for genetic heterogeneity. While duplications on either 17p13.3 or 10q24 [10] are the most frequent genetic cause, SHFM can be also associated with coding and non-coding mutations at other loci. Indeed, SVs involving the DYNC1I1 locus where regulatory elements for DLX5 and DLX6 are localized [11] , and mutations in TP63 , DLX5 , or WNT10B [12] have been previously associated with SHFM. The common underlying patho-mechanism of these mutations is thought to be the failure to maintain a proliferation/growth signal from the apical ectodermal ridge (AER), a signalling center of ectodermal cells at the distal end of the limb bud [13] . SHFM is also a clinically heterogeneous disease [14] . There is a high degree of clinical variability in individuals with SHFM-associated SVs even in the same family [15] , [16] . In addition, there can be high variability within affected individuals suggesting stochastic and other complex patho-mechanism that are not merely associated with gene dosage alteration. Tandem duplications on chromosome 10q24 at the LBX1 / FGF8 locus are considered the cause for SHFM type 3 (SHFM3) [15] , but the specific patho-mechanism of SHFM3-associated duplications remains unsolved. The reported duplications are at least 500 kb in size, encompassing five genes of the locus ( LBX1 , BTRC , POLL , DPCD , and FBXW4 ) but excluding the neighbouring FGF8 (Supplementary Fig. 1 ) [17] . While LBX1 is essential for early muscle cell differentiation and migration [18] , FGF8 is expressed in the AER together with other FGFs where it functions as a growth factor for the underlying mesechyme [19] . BTRC is part of the E3 ubiquitin-protein ligase complex which mediates the ubiquitination and subsequent proteasomal degradation of target proteins [20] , DPCD is involved in the generation and maintenance of ciliated cells [21] , POLL encodes for a DNA polymerase [22] , whereas FBXW4 is also involved in ubiquitin-mediated protein degradation [23] . Duplications can have different effects on gene regulation depending on their relative position to chromatin domain boundaries. Studies of the SOX9 locus, for example, have shown that duplications within the SOX9 TAD can lead to SOX9 mis/overexpression and sex reversal, whereas duplications that include the SOX9/KCNJ2 boundary and the KCNJ2 gene result in KCNJ2 misexpression and brachydactyly [4] . In the latter situation, a neo-TAD is formed leading to contact of the SOX9 enhancers with the KCNJ2 promoter and KCNJ2 expression in a SOX9-like pattern. Given these examples, it is conceivable that the SHFM3-associated duplications may have specific regulatory effects that could result in gene misexpression. In addition to the SHFM3 duplications at the LBX1 / FGF8 locus, we reported here a new case of SHFM3 malformation associated with an inversion at the same locus. This inversion was also of particular interest as the patient is a good example of clinical heterogeneity of this limb malformation within the same individual (Supplementary Fig. 2 ). To uncover the molecular mechanism underlying this congenital disease, we engineered a duplication and the inversion at the Lbx1/Fgf8 locus in mice using CRISPR/Cas9 genome editing tool [24] . While only the inversion led to a digit phenotype in mice, both SVs induced similar molecular phenotypes. Chromosome conformation capture Hi-C (cHi-C) analysis of the mouse developing limbs in mutants showed that both SVs led to a disruption of the wild-type three-dimensional chromatin configuration of the locus and ectopic enhancer-promoter contacts. Strikingly, this caused misexpression of two genes, Lbx1 and Btrc , in an Fgf8 -like pattern in the AER. Here, we show the impact of SVs at the Lbx1/Fgf8 locus on chromatin architecture and gene regulation and reveal the complex molecular patho-mechanism underlying SHFM3 limb malformation. With the emergence of novel sequencing technologies and the improvement in the discovery and characterization of SVs, this study illustrates the myriad ways by which SVs can cause disease (i.e., a combination of enhancer repositioning and gene misexpression), highlighting the challenging task of their interpretation in the clinic. SHFM3-associated SVs include TAD boundary and Fgf8 enhancers To characterize the 3D conformation at the Lbx1 / Fgf8 locus during mouse development, we performed cHi-C in wild-type murine limb buds at E11.5, a developmental stage where both Lbx1 and Fgf8 limb developmental genes are expressed (Fig. 1a ). We observed that the locus is characterized by the presence of a major chromatin loop (Fig. 1a , top dashed circle and double dashed lines) comprising two distinct smaller chromatin regulatory domains (Fig. 1a , single dashed lines). The centromeric and the telomeric domains contain the Lbx1/Btrc and the Fbxw4 / Fgf8 genes, respectively, and are hereafter referred to as Lbx1 and Fgf8 TADs (Fig. 1a ). These two domains are separated from neighbouring TADs and each other by CTCF-associated TAD boundaries in the classical divergent orientation [25] (Fig. 1a ). Poll and Dpcd are located within the boundary region separating Lbx1 and Fgf8 TADs and their expression might also contribute to the boundary. Given the divergent roles and expression pattern of Lbx1 and Fgf8 during limb development [26] , [27] (Fig. 1a ), separated regulatory domains can be expected to ensure correct gene regulation. The Fgf8 TAD contains several well characterized enhancers with AER-specific activity as well as other tissue-specific enhancers corresponding to the Fgf8 expression pattern in the embryo, such as the branchial arches, the somites, and the midbrain-hindbrain boundary [28] , [29] . Interestingly, all identified AER enhancers [28] are located within a 40 kb region in the introns of Fbxw4 (58, 59, 61, 66; yellow ovals in Fig. 1a ), with the exception of one enhancer (80; orange oval in Fig. 1a ) which is located in close proximity to Fgf8 . Fig. 1: Engineering of the SHFM-associated structural variations at the Lbx1 / Fgf8 locus. a cHi-C (data are shown as merged signal of n = 3 biological and 1 technical replicates) of extended Lbx1 / Fgf8 locus generated from wild-type E11.5 mouse limb buds. Lbx1 and Fgf8 are located within distinct TADs (indicated by single dashed lines) separated by boundaries (indicated by red hexagons) in correlation with CTCF binding sites, as indicated in ChIP-seq from E11.5 mouse limb buds [61] below. Loops (dashed circles) indicate interaction between CTCF sites. Interaction plots using virtual 4C from Fgf 8 and Lbx1 viewpoints (VP) are shown below. Regions of interactions relative to Lbx1 and Fgf8 within their own TADs are highlighted in yellow, whereas contacts with the boundary region between Lbx1 and Fgf8 TADs and those over such boundary are in violet and pink, respectively. Published Fgf8 enhancers [28] are indicated by ovals. Yellow ovals highlight enhancers driving Fgf8 expression in the AER and localized within the introns of Fbxw4 , while in orange is the only AER enhancer in close proximity to Fgf8 . b Schematic of human SHFM3 related structural variations (SVs). Red and blue lines in the duplications bar represent the different centromeric and telomeric breakpoints, respectively. Breakpoints of the inversion are shown below. c Schematic of the SHFM-associated SVs engineered in mice using CRISPR/Cas9 genome editing tool, particularly one selected tandem duplication ( Dup ) and the inversion ( Inv1 ). d Skeletal analysis of fore- and hindlimb stained with alcian blue (cartilage) and alizarin red (bone), from wild-type, heterozygous and homozygous Dup and Inv1 18.5 embryos. No particular phenotype was observed in both heterozygous and homozygous Dup and in heterozygous Inv1 , whereas fused bones and split digits were detected in homozygous Inv1 forelimbs. Full size image Virtual 4C analysis with viewpoints on Lbx1 and Fgf8 further emphasized how the interactions of these genes are to a large extend restricted to their respective regulatory domains (interactions are highlighted in yellow in Fig. 1a ). Virtual 4C demonstrates the specific domains of interaction but also shows a domain of overlapping interaction at the TAD boundary region (highlighted in violet in Fig. 1a ). Despite being two separate domains, the Lbx1 and Fgf8 TADs are also connected via an additional loop (Fig. 1a , top dashed circle in cHi-C map). This interaction is also visible in our 4C analysis (highlighted in pink in Fig. 1a ) suggesting that subpopulations of limb bud cells might have different configurations. This suggests a certain degree of leakiness of the Lbx1/Fgf8 boundary, leading to a level of intermingling of the two domains despite the very different expression patterns of Lbx1 and Fgf8 . Mapping of in-house and already published SHFM3 duplications onto the 3D structure of the locus showed that they all include the boundary between the Lbx1 and Fgf8 TADs (Fig. 1b ). Furthermore, all duplications comprised Lbx1 at the centromeric side and the previously identified Fgf8 AER enhancers located within Fbxw4 [29] , while excluding Fgf8 at the telomeric side (Fig. 1b and Supplementary Fig. 1 ). Mapping of the new SHFM-associated inversion showed that the boundary region between the Lbx1 and Fgf8 TADs and the Fgf8 AER enhancers are located within the inversion breakpoints, suggesting a potential common patho-mechanism. To investigate the effect of the SHFM3-associated duplications and inversion on chromatin configuration, gene expression, and phenotype, we engineered a human SHFM3 duplication ( Dup ) and the newly reported inversion ( Inv1 ) in mice (Fig. 1c ). Inv1 but not Dup results in a SHFM-like phenotype First, we analysed the mutant mice for skeletal phenotypes at developmental stage E18.5. In both heterozygous and homozygous Dup and in heterozygous Inv1 we did not observe any skeletal malformations in the extremities of all the analysed embryos ( n = 4 for Dup het, n = 5 for Dup hom and n = 8 for Inv1 het) (Fig. 1d ). Furthermore, none of the >25 adult mice with those genotypes from the established Dup and Inv1 mouse lines displayed a visible morphological phenotype. However, 3 out of 11 E18.5 homozygous Inv1 embryos exhibited skeletal defects with a tendency to digit separation and partially missing or fused digits/bones (Fig. 1d ), resembling the phenotype of SHFM patients [15] and particularly that of the SHFM3 inversion individual (Supplementary Fig. 2 ). Additionally, all homozygous Inv1 mutants showed underdeveloped forelimbs and hindlimbs (Supplementary Fig. 3a ). This latter phenotype is highly similar to the Fgf8 conditional knock-out [27] , [30] , suggesting that the expression of Fgf8 in the developing limb might be affected in the Inv1 homozygous mutants. Loss of Fgf8 expression is known to affect the proper development of humerus, radius, ulna, and to cause loss mainly of the first digit [27] , an overall phenotype different from SHFM3 based on the clinical cases reported so far in literature [9] , [15] , [17] . SHFM3-associated SVs result in ectopic 3D interactions The phenotype observed in the homozygous Inv1 mutants and the phenotypic discrepancy between the two types of SHFM3 SVs prompted us to study the effect on 3D genome organization during limb development. We thus performed cHi-C in homozygous Dup and Inv1 E11.5 murine limb buds (Fig. 2 ). Compared to wild-type (Fig. 2a ), the cHi-C map of the Dup mutant (Fig. 2c ) showed a general increase in the frequency of interactions within the duplicated region, reflecting the copy number increase. In the subtraction map ( Dup versus wild-type), the effect of the higher copy number on the signal intensity is corrected (Fig. 2c , mirror view). Interestingly, we observed a stripe of increased interactions (indicated by black arrowheads) involving the part of the Fgf8 TAD containing the Fgf8 AER enhancers comprised in the duplication (blue bar in Fig. 2c ) and a region immediately upstream of the Lbx1 centromeric TAD boundary (orange bar in Fig. 2c ). This reflected the formation of a neo-TAD, as illustrated in the schematic of the predicted linear configuration (Fig. 2d ). We also observed increased contacts between the entire Lbx1 TAD and the Fgf8 AER enhancers region (indicated by dashed rectangle and asterisks in Fig. 2c ). These interactions were established by the Fgf8 AER enhancers from the neo-TAD, with the endogenous and/or the duplicated Lbx1 TADs (Fig. 2d ). Indeed, in the Dup mutant, interactions between the Fgf8 AER enhancers and the telomeric duplicated Lbx1 TAD is favoured by a shorter distance, particularly with Lbx1 gene (~130 kb in Dup versus ~380 kb in wild-type configuration), and by the presence of a weaker TAD boundary (two CTCF binding sites instead of four). Moreover, the Fgf8 AER enhancers could also contact the centromeric endogenous Lbx1 TAD due to the previously mentioned leakiness of the boundary and the absence of their target gene Fgf8 , making these enhancers free to interact with the neighbouring Lbx1 gene and the entire Lbx1 TAD. Fig. 2: Ectopic 3D interactions upon structural rearrangements at the Lbx1 / Fgf8 locus. a Wild-type E11.5 mouse limb buds cHi-C (merged signal of n = 3 biological and 1 technical replicates). Red hexagons indicate boundaries, dashed circles highlight boundaries interactions. CTCF binding sites orientation and schematic of the locus are below. Yellow ovals highlight Fgf8 AER enhancers. b Schematic of the wild-type configuration. Lbx1 TAD in yellow, Fgf8 TAD in blue. Red squares highlight boundaries interactions. CTCF binding sites orientation, interactions between convergent CTCF and schematic of the locus are below. c cHi-C (merged signal of n = 3 biological and 1 technical replicates) of homozygous Dup E11.5 mouse limb buds. Subtraction map between wild-type and Dup interactions is shown in mirror view. Dashed circles indicate positions of preserved wild-type boundaries interactions, black arrow highlight the new contact reflecting the duplication breakpoints. Black arrowheads indicate gain of contacts between the region containing the Fgf8 AER enhancers (blue bar in the locus schematic below) and the region flanking the centromeric side of the Lbx1 TAD boundary (orange bar). Asterisks highlight the rectangular dashed area showing increased interactions between the Fgf8 AER enhancers region and the Lbx1 TAD. d Schematic of the predicted linear Dup configuration. The entire Lbx1 TAD is duplicated, remaining unchanged in its content and configuration, like the telomeric Fgf8 TAD. Between the two Lbx1 TADs, a neo-TAD forms. Below is a zoom-in view with red dashed arrows indicating potential ectopic contacts. e cHi-C (merged signal of n = 3 biological and 1 technical replicates) of homozygous Inv1 E11.5 mouse limb buds. Dashed circles indicate the positions of the original wild-type boundaries interactions, two (centromeric and telomeric) lost upon inversion. The inverted boundary is shown as blurry. Dashed lines on the right point out the new smaller Fgf8 TAD. Black arrowhead highlights the bow tie configuration representative of inverted regions. Black asterisks highlight the rectangular dashed area showing ectopic interactions between the Fgf8 AER enhancers region and the Lbx1 TAD, white asterisk points out the loss of interactions between Fgf8 and its AER enhancers. f Schematic of the Inv1 configuration with zoom-in of the locus highlighting potential ectopic interactions (red dashed arrows). Full size image Ectopic interactions between the Fgf8 AER enhancers region and the Lbx1 TAD were also observed for the Inv1 mutant (Fig. 2e,f ). In the inversion, the boundary between Lbx1 and Fgf8 TADs functioned as an anchor point around which part of the Fgf8 TAD was moved into the Lbx1 TAD and vice versa. Since the centromeric breakpoint of the inversion is relatively close to the boundary, the Lbx1 TAD was enlarged while the Fgf8 TAD was reduced in size. As a consequence, the Fgf8 AER enhancers were now relocated in the Lbx1 TAD resulting in increased contacts (dashed rectangle and black asterisks in Fig. 2e ) with the repositioned Fgf8 AER enhancer region, similar to our finding in the Dup . As a consequence of the reconfiguration of the locus, Fgf8 was now isolated from its AER enhancers and we indeed observed a loss of interactions between these elements and their endogenous gene (dashed rectangle with white asterisk in Fig. 2e ). Since the SHFM3 phenotype in humans manifests already in heterozygosity, we analysed the 3D chromatin configuration in Dup and Inv 1 het embryos and detected the same ectopic interactions as in homozygosity, but with lower frequency (Supplementary Fig. 3b, c ). Given that the overall configuration of the locus with two main TADs is conserved in humans (Fig. 3a ), we then investigated whether the observed interaction changes were also present in SHFM3 patients. We performed 4C-seq experiments in human fibroblasts from a patient carrying the SHFM3 duplication (fibroblasts from the inversion case were not available) and exhibiting the classical SHFM phenotype. We detected an increased interaction between the 125 kb region of FGF8 TAD containing the AER enhancers and both LBX1 and BTRC genes compared to healthy control (Fig. 3b ). This effect appeared to be specific as the 4C signal remained unchanged when using the viewpoint of FGF8 or when focusing on a region outside of the FGF8 TAD (Fig. 3b and Supplementary Fig. 4a ). As we showed that mouse virtual 4C is a good way of similarly quantifying cHi-C data (Fig. 1a ), we used it for the Dup and the Inv1 mouse mutants. We confirmed that the same ectopic interactions as in the patient data existed in the Dup mutants (Fig. 3c, d and Supplementary Fig. 4b ), indicating the applicability of our mutant mouse model for SHFM3. While a similar interaction between Lbx1/Btrc and the 125 kb AER enhancers region was present in the Inv1 mutant, we also observed ectopic interactions between Lbx1/Btrc and the Fgf8 gene that were specific to this mutant (Fig. 3c, d and Supplementary Fig. 4b ). We also detected a decreased interaction between Fgf8 promoter and its enhancer region, again suggesting Fgf8 expression might be affected in the Inv1 mutant (Fig. 3c, d ). Fig. 3: 4C-seq in SHFM3 patient fibroblasts reveals ectopic interactions involving LBX1 and BTRC , further supported by virtual 4C in mouse. a Hi-C at the LBX1 / FGF8 locus (hg19; chr10:102,668,128-103,840,922) derived from GM12878 cell [50] . TADs structures are similar between human and mouse. CTCF ChIP-seq from GM12878 cells [62] , [63] , orientation of CTCF binding sites and schematic of the human LBX1/FGF8 locus are shown below. Red arrow indicates a CTCF binding site in antisense orientation at the LBX1 centromeric TAD boundary present in mouse but not in human. Below is the normalized 4C-seq of human fibroblasts healthy control (grey) versus a SHFM3 patient carrying the duplication (green line) with viewpoints (VP) on FGF8 , LBX1 and BTRC promoters. Data are shown as merged signal of n = 2 replicates. b (Left panel) 4C-seq integrated signal over a 125 kb region comprising the FGF8 regulatory elements that are duplicated. (Right panel) A zoom-in view from the 4C-seq showing the region used for the integrated signal (blue rectangle). We observed an increase of contacts between both LBX1 and BTRC promoters and the FGF8 regulatory elements which is not present in control regions (Supplementary Fig. 4 ). c Similar representation as in ( a ) showing the mouse CTCF and virtual 4C (generated from E11.5 limbs cHi-C maps from Fig. 2 ) tracks. Wild-type (WT) signal is shown in grey and Dup and Inv1 with a green and orange line, respectively. Data are shown as merged signal of n = 3 replicates. d (Left panel) Virtual-4C integrated signal over the 125 kb region comprising Fgf8 regulatory elements that are affected by the duplication and the inversion. (Right panel) A zoom-in view from the virtual-4C showing the 125 kb used for the integrated signal (blue rectangles). Black arrow highlights a gain of contact observed only for Lbx1 view point with the Fgf8 gene, outside of the region of interest. Gain of interactions is observed between both Lbx1 and Btrc promoters and the Fgf8 regulatory elements which is not present in control regions (Supplementary Fig. 4 ). Full size image Dup and Inv1 lead to Lbx1 and Btrc misexpression in the AER The 3D conformation data were not sufficient to explain the discrepancy of morphological phenotype between the Inv1 and Dup mutants. To investigate the effect of the observed chromatin rearrangements on gene expression and possibly link it to the observed phenotype, we performed detailed expression analysis (RNA-seq, single-cell RNA-seq and whole mount in situ hybridisation (WISH)) at developmental stage E11.5. In the Dup hom mutant, all genes within the duplication ( Lbx1 , Btrc , Poll , Dpcd and Fbxw4 ) were significantly upregulated in the developing limb buds, corresponding to the copy number increase (Fig. 4a and Supplementary Data 1 ). In the Inv1 hom mutant, Fbxw4 and Fgf8 were downregulated, reflecting the disruption of the Fbxw4 and the repositioning of the Fgf8 AER enhancers to the neighboring Lbx1 TAD (Fig. 4a and Supplementary Data 1 ). Strikingly, Lbx1 and Btrc exhibited increased expression levels in the Inv1 mutant, indicating that the observed chromatin rearrangement had an effect on gene expression. Genes outside of the Fgf8 and Lbx1 TADs ( Sif2 , Twnk and Oga ) remained unchanged in both Dup and Inv1 mutants (Fig. 4a ). Fig. 4: Dup and Inv1 chromatin rearrangements have an impact on gene expression. a Bar plot representing the rpkm value normalized to wild-type for genes in the Lbx1 and Fgf8 TADs and flanking genes ( Slf2 and Twnk (centromeric), Oga (telomeric)) from RNA-seq data of homozygous Dup and Inv1 E11.5 limb buds. n = 2 biological replicates per condition. Schematic of the locus shows the position of the genes, the TAD boundaries (red hexagons) and the parts included in the Dup and the Inv1 mutants. Wild-type Dup and Inv1 samples are shown in black, green and orange, respectively. b Uniform manifold approximation and projection (UMAP) showing 8 cell clusters identified via scRNA-seq of E11.5 mouse limbs from wild-type, Dup and Inv1 mutants ( n = 1). c Violin plot representing the normalized expression of the 6 genes at the locus in AER, dorso-ventral (DV) ectoderm, mesenchyme and myocytes from E11.5 hindlimbs. The Dup mutant (green) was generated in a C57Bl6 background and thus compared to a C57Bl6 wild-type sample (dark grey) whereas the Inv1 mutant (orange) was generated in a G4 (129sv x C57Bl6) and compared to a G4 wild-type sample (light grey). Full size image To investigate whether these changes of gene expression were specific to certain regions of the limb bud, we performed single-cell RNA-seq (scRNA-seq) from E11.5 wild-type, Dup hom and Inv1 hom limb buds. Individual clusters corresponding to the major cell types in the developing limb were identified including mesenchyme, dorso-ventral ectoderm, AER and muscle as well as satellite cell types such as neurons, lymphocytes, keratinocytes and endothelial cells (Fig. 4b and Supplementary Fig. 5a–c ). In wild-type limbs, Fgf8 expression was only present in the AER and Lbx1 was expressed only in muscle cells whereas Btrc was expressed at a low level in all limb cells with higher expression in the AER (Fig. 4c ). The three other genes of the locus were expressed in all major cell types of the developing limb at a rather low level (Fig. 4c ). The single-cell data were in agreement with the bulk RNA-seq such that the five genes included in the duplication ( Lbx1, Btrc, Poll, Dpcd and Fbxw4 ), but not Fgf8 , displayed increased expression in the Dup mutant compared to wild-type (Fig. 4c ). The loss of Fgf8 expression in the Inv1 mutant was also confirmed. Interestingly, in the AER, both Lbx1 and Btrc showed a stronger increase of expression in the Dup mutant compared to wild-type than what we would expect with the increased copy number, indicating misexpression in the AER. In the Inv1 mutant, where no copy number changes occurred, we observed the misexpression to be even stronger (Fig. 4c and Supplementary Fig. 5d ), particularly for Btrc . These results suggested that both Lbx1 and Btrc were activated by the Fgf8 AER enhancers now able to contact the two genes’ promoters (Fig. 3d ). Thus, the scRNA-seq data confirmed the bulk RNA-seq data and showed, in addition, that Lbx1 and Btrc were misexpressed in the AER with a stronger effect in the Inv1 . Next, we performed WISH to confirm and further investigate potentially altered expression patterns. We confirmed that Lbx1 , normally expressed in migrating muscle cells (black arrowheads for Lbx1 in Fig. 5a ), and Btrc were ectopically expressed in the AER, in both homozygous (Fig. 5a ) and heterozygous (Supplementary Fig. 6a ) Dup and Inv1 E11.5 embryos. As observed in the scRNA-seq data, an even more pronounced misexpression of both genes was also observed in the Inv1 hom mutants (Fig. 5a ). In the Dup mutant, Fgf8 expression was unchanged compared to wild-type. In contrast, in the Inv1 mutant we confirmed a complete loss of Fgf8 expression in homozygosity (Fig. 5a ) and a partial loss in heterozygosity (Supplementary Fig. 6a ), likely due to the loss of the endogenous interactions of Fgf8 with its enhancers. Finally, we did not detect any misexpression in the AER for Poll , Dpcd and Fbxw4 , neither in Dup , nor in the Inv1 mutants (Supplementary Fig. 6b ). Fig. 5: Ectopic interactions result in Lbx1 and Btrc misexpression in the AER. a Whole-mount in situ hybridization for Fgf8 , Lbx1 and Btrc at E11.5. Expression was checked and confirmed in at least 3 or more homozygous embryos (at least n = 3 biological replicates). b Schematic of the Lbx1 / Fgf8 locus for CRISPR/Cas9 Fgf8 AER enhancer KI allele. Yellow ovals highlight Fgf8 AER enhancers. c GO analysis for the MGI Mammalian phenotype enrichment terms [59] using the top 200 genes that are up-regulated genes in the Dup mutant compared to wild-type in the AER cells from the scRNA-seq data. The 5 most significant enriched terms are represented on a -log10 ( p -value) scale. P -value was computed using a Fisher exact test. d Heatmap showing the expression of 6 genes ( Lbx1, Myog, Gab1, Rela, Mapk14 and Dnm2 ) associated with the myogenic enriched terms in ( c ) in the AER cells. Each column represents one AER cell and the z-score scaled expression is indicated for each gene, showing a global increased expression in the Dup mutant’s AER cells. Full size image Our findings suggest that the four previously described Fgf8 AER enhancers are the main regulators of Fgf8 expression in this tissue [28] , [29] . To confirm that, we used CRISPR/Cas9 technology to delete those four enhancers (CE58, CE59, CE61 and CE66) in a wild-type background (Δ Fgf8 -AER-enh, Supplementary Fig. 7a ) and compared the outcome to what we observed in the Inv1 E11.5 embryos. Fgf8 expression appeared to be strongly affected in both mutants (Supplementary Fig. 7b–c ), resulting in a similar reduction of limb bud size (Supplementary Fig. 7c ). Lbx1 and Btrc expression was not affected in the Δ Fgf8 -AER-enh mutant. Knowing that these enhancers control the majority of Fgf8 expression in the AER, we tested whether the repositioning of the AER enhancers was sufficient to induce ectopic expression of Btrc and Lbx1 in the AER. We used CRISPR/Cas9 technology to insert the four Fgf8 AER enhancers in the Lbx1 TAD in a wild-type background ( Fgf8 AER enh KI , Fig. 5b ). Given the presence of a CTCF binding site within enhancer CE58 and our aim to not create any new boundary upon knock-in we removed the CTCF recognition motif from enhancer CE58. WISH of Fgf8 AER-enhancer KI E11.5 mutant embryos showed misexpression of Lbx1 and Btrc in the AER (Fig. 5a ), supporting the ability of the Fgf8 enhancers to activate other genes. Of note, we observed that Lbx1 was ectopically expressed in the AER of all analysed embryos, while Btrc was present in the AER of 50% of the examined embryos and displayed a much lower signal. Importantly, this result further confirmed that the observed ectopic expression of Lbx1 and Btrc in the AER in the Dup and Inv1 mutants was due to activation by Fgf8 enhancers. Lbx1 AER misexpression is associated with myogenic signature We and others have previously shown that ectopic gene expression during organ formation can lead to developmental malformation [3] , [4] , [31] , [32] , [33] . However, the molecular consequences of the observed misexpression are still unknown. In both mutants, Lbx1 is part of the top 3 up-regulated genes in the AER (Supplementary Data 2 ). We reasoned that Lbx1 could activate its gene regulatory network in the AER and to investigate this we performed a Gene Ontology (GO) search using the 200 genes most differentially up-regulated in the AER cells in Dup and Inv1 compared to wild-type (C57Bl6 and G4, respectively) hindlimb (Supplementary Data 2 ). Strikingly, using the MGI mammalian phenotype terms, 4 out of the 5 and 3 out of the 10 most enriched terms in the Dup and Inv1 comparison respectively, were related to myogenic phenotypes (Fig. 5c and Supplementary Fig. 6c ). Genes associated with these terms included Lbx1 , Myog, Gab1, Rela, Mapk14 and Dnm2 which were all expressed at a higher level in more cells in the AER of the Dup mutant compared to wild-type (Fig. 5d ). Additionally, expression of one of the genes, Myog , was also significantly increased in the bulk RNA-seq differential analysis data from limb buds from the Inv1 mutant (Supplementary Data 1 ). Of note, Lbx1 expression was detectable in almost all AER cells while none of the wild-type AER cells expressed Lbx1 , corroborating our previous observations. Overall, it suggested that gene misexpression could trigger a specific pathway. Regarding the effect of Btrc misexpression, despite this gene being strongly misexpressed in the AER in Inv1 mutant, the downstream effect of an E3 ubiquitin ligase would be expected to be seen at the protein level and unlikely at the mRNA level [34] . SHFM-like phenotype requires Lbx1 and Btrc AER misexpression To further investigate the contribution of Lbx1 and Btrc to SHFM, we engineered two more CRISPR/Cas9 alleles to promote Lbx1 or Btrc misexpression alone in the AER and compared it to Dup and Inv1 where genes were simultaneously misexpressed. First, we generated a second, slightly larger inversion ( Inv2 ) including the Fgf8 AER enhancers and Btrc (Fig. 6a ). This mutant showed ectopic interactions between the Fgf8 AER enhancers and Lbx1 only, as observed in cHi-C and particularly in the subtraction cHi-C map (Fig. 6b ) but in general with much lower intensity compared to Inv1 mutant. Misexpression of only Lbx1 but not Btrc was indeed detected in the AER (Fig. 6D ). We also noticed that the embryos exhibited underdeveloped head structure, most likely as a consequence of the midbrain-hindbrain boundary Fgf8 enhancers [28] , [29] (CE64 and CE79, see Fig. 1a ) being repositioned outside of the Fgf8 TAD in Inv2 . To investigate the effect of an ectopic expression of Btrc alone, we re-targeted the Inv1 allele and deleted Lbx1 ( Inv1 ∆Lbx1 ) (Fig. 6a ). As expected, no misexpression for Lbx1 was detected in the AER and in the limb in general, while Btrc was transcriptionally active (Fig. 6d ). In addition, we observed a weak expression of Fgf8 rescued in the AER, underlining the ability of the Fgf8 AER enhancers to re-contact their endogenous target gene in the absence of Lbx1 and, similar to the situation in the Dup mutant. Skeletal analysis of Inv2 and Inv1 ∆Lbx1 homozygous mutants (Fig. 6e ) revealed underdeveloped limbs due to a complete ( Inv2 ) or strong ( Inv1 ∆Lbx1 ) loss of Fgf8 expression (Fig. 6d ), but none of them ( n = 10 for Inv2 and n = 7 for Inv1 ∆Lbx1 ) showed the level of SHFM phenotype observed in Inv1 (Fig. 1d ), supporting the notion that misexpression of both Lbx1 and Btrc is required to develop the SHFM-like phenotype. Furthermore, the comparison of Inv1 , Inv2 and Inv1 ∆Lbx1 indicated that the level of Fgf8 expression might have a role in triggering the SHFM-like phenotype in combination with Lbx1 and Btrc misexpression. The Inv2 phenotype, where Fgf8 expression was completely lost, seemed indeed more severe than Inv1 ∆Lbx1 , where Fgf8 was only partially lost (Fig. 6e and Fig. 7 ). Fig. 6: Misexpression of both Lbx1 and Btrc is required to develop a SHFM phenotype. a Schematics of the Lbx1 / Fgf8 locus for CRISPR/Cas9 Inv2 and Inv1 ∆Lbx1 alleles. Yellow ovals highlight Fgf8 AER enhancers. b cHi-C (data are shown as merged signal of n = 3 biological and 1 technical replicates) of homozygous Inv2 from E11.5 mouse limb buds. The subtraction map between wild-type and Inv2 interactions is shown in mirror view. Dashed circles indicate the position of the original wild-type interactions between boundaries, two of them lost upon reshuffling of the boundary between Lbx1 and Fgf8 TADs as a consequence of this inversion. The boundary involved in the inversion is shown as blurry. Black arrowhead highlights the bow tie configuration representative of the inverted regions. The rectangular dashed area highlighted by black asterisks show ectopic interactions compared to wild-type between the Fgf8 AER enhancers region and the one containing now only Lbx1 and not anymore Btrc . White asterisks point out the loss of interactions between Fgf8 and its AER enhancers. c Schematic of Inv2 configuration. Upon this inversion, the Fgf8 AER enhancers are repositioned within a smaller Lbx1 TAD, whereas the Fgf8 TAD is increased in size due to the inversion of the boundary and contains now Btrc , isolated from the Fgf8 AER enhancers. Below is a zoom-in of the locus highlighting the potential ectopic interactions (red dashed arrow) involving the Fgf8 AER enhancers now repositioned within the Lbx1 TAD. d Whole-mount in situ hybridization for Fgf8 , Lbx1 and Btrc at E11.5. Expression was checked and confirmed in at least 3 or more homozygous embryos (at least n = 3 biological replicates). e Skeletal analysis of E18.5 limbs stained with alcian blue (cartilage) and alizarin red (bone). Hands and feet from wild-type, Inv2, Inv1 ∆Lbx1 and Fgf8 AER enhancer KI E18.5 embryos. At least n = 3 biological replicates. Full size image Fig. 7: Combinatorial effects on gene expression at the Lbx1 / Fgf8 locus leads to SHFM3 digit fusion phenotype. Schematic overview of the Lbx1-Fgf8 TADs (top) and Lbx1 , Btrc and Fgf8 expression in the developing limb at E11.5 and skeletal phenotype at E18.5 among the different structural rearrangements (bottom). Yellow and violet patterns represent endogenous expression in the limb bud and misexpression in the AER of Lbx1 and Btrc , respectively. Turquoise pattern highlights Fgf8 expression in the AER. Ectopic expression of both Lbx1 and Btrc in the AER is observed for the Dup , Inv1 and Fgf8 AER enhancer KI ( Fgf8 AER enh KI ) mutant embryos at E11.5. However, only the Inv1 mutants, for which the level of Lbx1 and Btrc expression in the AER is higher and Fgf8 expression is missing, show a digit fusion phenotype at E18.5, reminiscent of human SHFM. Ectopic expression of either Lbx1 alone ( Inv2 mutant) or Btrc alone ( Inv1 ΔLbx1 mutant) together with complete ( Inv2 ) or partial ( Inv1 ΔLbx1 ) loss of Fgf8 AER expression is not enough to lead to the digit fusion SHFM-like phenotype but only results in an Fgf8 -KO limb phenotype. Full size image Finally, the level of Lbx1 and/or Btrc misexpression is likely to also play a role in the manifestation of the limb phenotype. Indeed, in the Dup and Fgf8 AER-enhancer KI mutants, the level of Btrc misexpression was lower than in the Inv1 mutant (Fig. 5a ) and no phenotype was detected (Fig. 1d and Fig. 6e ) despite misexpression of both Lbx1 and Btrc genes in the AER. Split-hand/foot malformation (SHFM) is a congenital limb malformation affecting the central rays of the hands and/or feet (OMIM #183600, #313350, #600095, #605289, and #606708). The condition is a classic example of allelic heterogeneity, phenotypic variability, and pleiotropy [35] . Here, we focused on SHFM type 3 which has been associated with rearrangement at the FGF8 / LBX1 locus. cHi-C of the Lbx1 / Fgf8 locus in mouse limb bud showed that the region consists of two major TADs, each harbouring an important developmental gene with strikingly different expression patterns (Fig. 7 ). The Fgf8 TAD contains a number of well-characterized enhancers that regulate Fgf8 specific expression in the AER and in other tissues [28] . The neighbouring TAD contains Lbx1 , a muscle-specific transcription factor expressed only in migrating muscle cells and Btrc , a ubiquitin ligase expressed at a low level in most limb cells and more stringently in the AER (Fig. 4c ). The two regulatory TADs are separated by a boundary with divergent CTCF sites. A combination of cHi-C and 4C analysis demonstrated that the two domains are connected via a larger loop between the centromeric Lbx1 TAD boundary and the telomeric Fgf8 TAD boundary, resulting in a certain degree of contact of one domain with the other across the boundary (Fig. 1a ). By re-engineering a human SHFM3-associated duplication in mice we observed ectopic interactions between the Fgf8 AER enhancers and two other genes in the locus, Lbx1 and Btrc . The same ectopic interactions were present in fibroblasts from a SHFM3 affected individual with duplication. In mice, this resulted in misexpression of Lbx1 and Btrc in the AER in a typical Fgf8 pattern. In contrast, Fgf8 expression remained unchanged. Indeed, Fgf8 was not included in the duplication and a fully intact Fgf8 regulatory landscape remained, ensuring normal expression. The duplication resulted in the formation of a neo-TAD [4] which consisted of the Fbwx4 gene and the Fgf8 AER enhancers but no other genes. Our results suggest that the neo-TAD by itself does not have any consequences, as no ectopic interactions between Fbxw4 and the Fgf8 AER enhancers and/or misexpression of Fbxw4 in the AER were detected (Fig. 2 and Supplementary Fig. 6b ). In a screen for structural variations in a cohort of patients with limb malformations, we also identified an inversion at the SHFM3 locus. Re-engineering of the human inversion in mice ( Inv1 ) showed that the inversion resulted in a shift of regulatory elements from the Fgf8 TAD into the Lbx1 TAD [5] thereby giving rise to the equivalent regulatory effect as the Dup . Interestingly, as for the duplication, the inversion involved the four essential Fgf8 AER enhancers (CE58, CE59, CE61, CE66) that are located in the introns of the Fbxw4 gene (Fig. 1a, b ). Previous experiments demonstrated that a loss of Fgf8 expression in the AER upon deletion resulted in similar defects as conditional ablation of Fgf8 in the limb [27] , [28] . In Inv1 we also observed a loss of Fgf8 expression and the corresponding Fgf8 loss of function phenotype. Thus, a repositioning of the boundary by the inversion was sufficient to disconnect Fgf8 from its enhancers resulting in a loss of Fgf8 expression similar to the 4 AER enhancers deletion (Supplementary Fig. 7 ). The effect of Inv1 was thus similar to the reported inversion at the Sox9/Kcnj2 locus which resulted in a loss of Sox9 expression due to a swap of Sox9 regulatory elements from the Sox9 TAD to the Kcnj2 TAD [36] . In both SHFM-associated rearrangements, only Lbx1 and Btrc were misexpressed in the AER. Poll , Dpcd and Fbxw4 showed very low levels of expression in these cells. This strongly suggests that these genes were not involved in the pathogenesis of SHFM3. Our conclusion that Lbx1 and Btrc were ectopically activated by the Fgf8 AER enhancers was further supported by the insertion of the AER enhancers in the Lbx1 TAD ( Fgf8 AER enh KI) . As in the duplication and in the inversion, the Fgf8 AER enhancers were able to activate both Btrc and Lbx1 , with the latter being more affected. In Inv1 the interactions were possible through the repositioning of the Fgf8 AER enhancers within the Lbx1 TAD similar to the Fgf8 AER enh KI mutant. In the Dup , the situation is more complex. Here, the duplicated Fgf8 AER enhancers are located within the neo-TAD but without their natural target promoter ( Fgf8 ). This situation likely results in increased contacts across the leaky Lbx1 / Fgf8 boundary on the centromeric side as well as the newly positioned boundary telomeric of the neo-TAD, as indicated by the dashed line in Fig. 2d . Thus, the common mechanism between the two SVs seems to be the ectopic expression of Btrc and Lbx1 in the AER driven by Fgf8 AER enhancers. To quantify the expression levels specifically in the AER, we performed single-cell RNA-sequencing of E11.5 limb buds. While the misexpression of Lbx1 was similar in both mutants, we detected a higher AER misexpression of Btrc in the Inv1 mutant compared to the Dup (Fig. 4c ). Interestingly, two studies have reported SHFM3 malformation in patients with smaller duplication containing only BTRC alone [37] or BTRC and POLL [38] , suggesting that abnormal expression of Btrc could be the main factor for the pathology of the human SHFM3 phenotype. Our data suggest that in mice, a high level of mis-expression of both Btrc and Lbx1 is required to generate the phenotype (Fig. 6 ). Finally, we cannot rule out the impact of genetic modifiers in different genetic backgrounds which might influence the manifestation of the phenotype, as observed in various congenital malformations such as for the role of TBX6 in scoliosis [39] . However, the precise pathomechanism through which Btrc and Lbx1 cause the phenotype is still unclear. The Dactylaplasia ( Dac ) mouse mutant displays a similar phenotype to the one observed in some SHFM3 patients and the two corresponding alleles ( Dac1j and Dac2j ) map to the region with the duplications and inversion in SHFM3 [40] . Based on these similarities, the mutant has long been thought as a model for human SHFM3, but Dac1j and Dac2j were shown to be associated with insertions of a MusD retrotransposon upstream of the Fbxw4 gene and within intron 5 of Fbxw4 , respectively [40] . The absence of any structural variations in these mutants and the differences between the nature of the human and mouse genomic abnormalities argue against a common pathogenesis. However, both the mouse and the human mutations involve the regulatory elements located within and around the Fbxw4 gene possibly providing a common pathogenetic mechanism. Similar to the reported misexpression of Pax3 in an Epha4 -like pattern in the limb in brachydactyly [3] , misexpression of the muscle-specific transcription factor Lbx1 and the ubiquitin ligase Btrc in the AER are likely to have effects on gene expression and thus the functionality of the AER. This interpretation is supported by our finding that Lbx1 misexpression is associated with the activation of muscle genes in the AER cells (Fig. 5c ). This effect seems to be stronger in the Dup , but given the low number of AER cells available for the differential expression analysis, we need to take this aspect with caution and consider the fact that other changes in gene expression could be stronger in Inv1 due to the lack of Fgf8 expression in this mutant. Btrc is part of a E3 ubiquitin-protein ligase complex which mediates the ubiquitination and subsequent proteasomal degradation of target proteins thereby participating in Wnt and BMP signalling [41] , both important signalling components of the AER. The ectopic expression of this ubiquitin ligase may thus contribute to cellular dysfunction in the AER. The AER is the major signalling center for proximodistal growth and distal limb development. It is induced and maintained through the reciprocal interactions between the ectoderm and the underlying mesenchyme involving Wnt-Bmp-Fgf signaling pathways [42] . Disruption or malfunction of the AER results in diminished growth and thus hypoplasia/aplasia of digits, correlating with the SHFM phenotype [43] . Our results support the concept that SHFM is caused by AER defects, and in SHFM3 by misexpression of Lbx1 and Btrc in the AER. Finally, we cannot exclude a potential contribution of a loss of Fgf8 expression to the Inv1 mutant phenotype. Mice are commonly used as a model organism to study human disease because of the similarities in genetics, physiology and organ development. However, inter-species differences exist and account for genotype-to-phenotype divergences between mouse and human [44] . When comparing CTCF binding sites in mouse and human at the FGF8 locus, we noticed that the centromeric Lbx1 TAD boundary is missing one binding site in reverse orientation in human in comparison to mouse (red arrow in Fig. 3a ). This additional binding site in mouse could thus interfere with the levels of ectopic interactions between the Fgf8 AER enhancers and Lbx1 and Btrc in the Dup mutant, consequently reducing the level of misexpression in the AER. Indeed, misexpression levels related to the rearrangements may explain the absence of a striking phenotype in the Dup in comparison to Inv1 which is associated with highest levels of Lbx1 and Btrc misexpression, causing a mouse phenotype similar to the human phenotype. Overall, this study offers insights into: i) the molecular phenotype of SHFM3-associated duplications and inversion, ii) gene regulation at the Lbx1 / Fgf8 locus in the context of 3D genome architecture and, iii) the consequences deriving from perturbations of the local chromatin structure. Notably, we provide a complex scenario by which SVs can cause disease. Indeed, we report in this study an example of SVs causing disease through a combined position effect mechanism resulting in ectopic gene misexpression involving multiple genes and a dose-dependent effect. To the best of our knowledge, the SVs-associated pathogenic mechanism reported in this study has not been shown previously. In the era of whole genome sequencing (WGS) and the increased number of detected SVs, the medical interpretation of SVs and the prediction of their phenotypic consequences remain unsatisfactory. Thus, this study provides a conceptual framework when interpreting the pathogenic potential of these variant types. The experiments were not randomized. The investigators were not blinded to allocation during experiments and outcome assessment. Ethical approvals All animal procedures were conducted as approved by the local authorities (LAGeSo Berlin) under license numbers G0243/18 and G0176/19. All animal experiments followed all relevant guidelines and regulations. The study design and conduct complied with all relevant regulations regarding the use of human participants and was conducted in accordance with the criteria set by the Declaration of Helsinki. Congenital limb malformations were observed at clinical genetic centres in Germany and in Italy. Given the nature of their phenotype, patients were offered additional diagnostic investigations in accordance with regulations for studies on human subjects at the respective centres. Informed consent to participate to the study and to publish clinical data was obtained from all patients (or their legal guardian). The study protocol was approved by the ethics committee at the Charité Universitätsmedizin Berlin, Germany. Mouse embryonic stem cell targeting Culture and genome editing of mouse embryonic stem cells (mESCs) was performed as described previously [24] , [36] . Briefly, G4 (129sv/C57Bl6 hybrid) mESCs were seeded on a monolayer of CD1 feeder cells and transfection was performed via FuGENE technology (Promega, Cat. #E5911) using 8ug of each CRISPR construct of interest delivered through the pX459 vector (which contains also a Puromycin-resistance cassette). After 24 h, cells were split onto DR4 Puromycin-resistant feeders and selection with Puromycin was carried on for 2 days. Resistant growing clones were then picked and grown into 96-well-plates on CD1 feeders. All clones were genotyped by PCR (Supplementary Table 2 ). 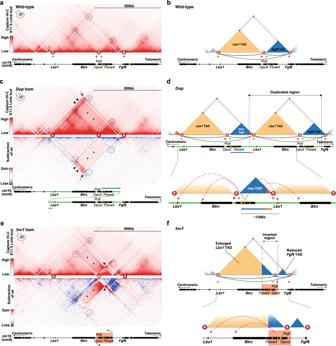Fig. 2: Ectopic 3D interactions upon structural rearrangements at theLbx1/Fgf8locus. aWild-type E11.5 mouse limb buds cHi-C (merged signal ofn= 3 biological and 1 technical replicates). Red hexagons indicate boundaries, dashed circles highlight boundaries interactions. CTCF binding sites orientation and schematic of the locus are below. Yellow ovals highlightFgf8AER enhancers.bSchematic of the wild-type configuration.Lbx1TAD in yellow,Fgf8TAD in blue. Red squares highlight boundaries interactions. CTCF binding sites orientation, interactions between convergent CTCF and schematic of the locus are below.ccHi-C (merged signal ofn= 3 biological and 1 technical replicates) of homozygousDupE11.5 mouse limb buds. Subtraction map between wild-type andDupinteractions is shown in mirror view. Dashed circles indicate positions of preserved wild-type boundaries interactions, black arrow highlight the new contact reflecting the duplication breakpoints. Black arrowheads indicate gain of contacts between the region containing theFgf8AER enhancers (blue bar in the locus schematic below) and the region flanking the centromeric side of theLbx1TAD boundary (orange bar). Asterisks highlight the rectangular dashed area showing increased interactions between theFgf8AER enhancers region and theLbx1TAD.dSchematic of the predicted linearDupconfiguration. The entireLbx1TAD is duplicated, remaining unchanged in its content and configuration, like the telomericFgf8TAD. Between the twoLbx1TADs, a neo-TAD forms. Below is a zoom-in view with red dashed arrows indicating potential ectopic contacts.ecHi-C (merged signal ofn= 3 biological and 1 technical replicates) of homozygousInv1E11.5 mouse limb buds. Dashed circles indicate the positions of the original wild-type boundaries interactions, two (centromeric and telomeric) lost upon inversion. The inverted boundary is shown as blurry. Dashed lines on the right point out the new smallerFgf8TAD. Black arrowhead highlights the bow tie configuration representative of inverted regions. Black asterisks highlight the rectangular dashed area showing ectopic interactions between theFgf8AER enhancers region and theLbx1TAD, white asterisk points out the loss of interactions betweenFgf8and its AER enhancers.fSchematic of theInv1configuration with zoom-in of the locus highlighting potential ectopic interactions (red dashed arrows). Positive clones were expanded, their genotyping further confirmed by PCR, qPCR (Supplementary Table 3 ) and Sanger sequencing of PCR products, and used for further experiments only if the successful modification could be verified. 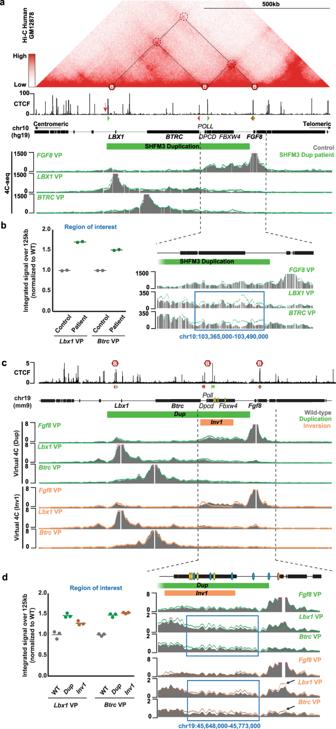Fig. 3: 4C-seq in SHFM3 patient fibroblasts reveals ectopic interactions involvingLBX1andBTRC, further supported by virtual 4C in mouse. aHi-C at theLBX1/FGF8locus (hg19; chr10:102,668,128-103,840,922) derived from GM12878 cell50. TADs structures are similar between human and mouse. CTCF ChIP-seq from GM12878 cells62,63, orientation of CTCF binding sites and schematic of the humanLBX1/FGF8locus are shown below. Red arrow indicates a CTCF binding site in antisense orientation at theLBX1centromeric TAD boundary present in mouse but not in human. Below is the normalized 4C-seq of human fibroblasts healthy control (grey) versus a SHFM3 patient carrying the duplication (green line) with viewpoints (VP) onFGF8,LBX1andBTRCpromoters. Data are shown as merged signal ofn= 2 replicates.b(Left panel) 4C-seq integrated signal over a 125 kb region comprising theFGF8regulatory elements that are duplicated. (Right panel) A zoom-in view from the 4C-seq showing the region used for the integrated signal (blue rectangle). We observed an increase of contacts between bothLBX1andBTRCpromoters and theFGF8regulatory elements which is not present in control regions (Supplementary Fig.4).cSimilar representation as in (a) showing the mouse CTCF and virtual 4C (generated from E11.5 limbs cHi-C maps from Fig.2) tracks. Wild-type (WT) signal is shown in grey andDupandInv1with a green and orange line, respectively. Data are shown as merged signal ofn= 3 replicates.d(Left panel) Virtual-4C integrated signal over the 125 kb region comprisingFgf8regulatory elements that are affected by the duplication and the inversion. (Right panel) A zoom-in view from the virtual-4C showing the 125 kb used for the integrated signal (blue rectangles). Black arrow highlights a gain of contact observed only forLbx1view point with theFgf8gene, outside of the region of interest. Gain of interactions is observed between bothLbx1andBtrcpromoters and theFgf8regulatory elements which is not present in control regions (Supplementary Fig.4). 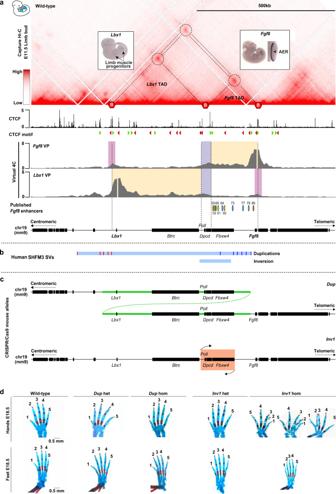qPCR results were analyzed using the QuantStudio 7 Flex Real-Time PCR Software (version 1.7.1, Applied Biosystems). The size and position of the human structural variations (hg19/GRCh37) were converted to the mouse genome (mm9/NCBI37) using the UCSC liftOver tool ( https://genome.ucsc.edu/cgi-bin/hgliftOver ). Fig. 1: Engineering of the SHFM-associated structural variations at theLbx1/Fgf8locus. acHi-C (data are shown as merged signal ofn= 3 biological and 1 technical replicates) of extendedLbx1/Fgf8locus generated from wild-type E11.5 mouse limb buds.Lbx1andFgf8are located within distinct TADs (indicated by single dashed lines) separated by boundaries (indicated by red hexagons) in correlation with CTCF binding sites, as indicated in ChIP-seq from E11.5 mouse limb buds61below. Loops (dashed circles) indicate interaction between CTCF sites. Interaction plots using virtual 4C fromFgf8 andLbx1viewpoints (VP) are shown below. Regions of interactions relative toLbx1andFgf8within their own TADs are highlighted in yellow, whereas contacts with the boundary region betweenLbx1andFgf8TADs and those over such boundary are in violet and pink, respectively. PublishedFgf8enhancers28are indicated by ovals. Yellow ovals highlight enhancers drivingFgf8expression in the AER and localized within the introns ofFbxw4, while in orange is the only AER enhancer in close proximity toFgf8.bSchematic of human SHFM3 related structural variations (SVs). Red and blue lines in the duplications bar represent the different centromeric and telomeric breakpoints, respectively. Breakpoints of the inversion are shown below.cSchematic of the SHFM-associated SVs engineered in mice using CRISPR/Cas9 genome editing tool, particularly one selected tandem duplication (Dup) and the inversion (Inv1).dSkeletal analysis of fore- and hindlimb stained with alcian blue (cartilage) and alizarin red (bone), from wild-type, heterozygous and homozygousDupandInv118.5 embryos. No particular phenotype was observed in both heterozygous and homozygousDupand in heterozygousInv1, whereas fused bones and split digits were detected in homozygousInv1forelimbs. A list of single guide RNAs (sgRNAs, designed using http://crispr.mit.edu/ platform) used for CRISPR/Cas9 genome editing is given in Supplementary Table 1 . For the Fgf8-AER-enh-KI mutant, a 6993 bp DNA fragment containing the 4 Fgf8 -AER enhancers with a deletion of the CTCF site in enhancer CE58 was synthetised and subsequently cloned into a pUC vector by Genewiz . Homology arms targeting the Lbx1 locus were then cloned using Gibson assembly and the resulting vector was transfected in mESCs together with the pX459-sgRNA for CRISPR/Cas9 homology-directed-repair (HDR). Generation of mice Mice were generated from genome-edited mESCs by diploid or tetraploid aggregation [45] and genotyped by PCR and qPCR analysis. Cells were seeded on CD1 feeders and grown for 2 days before aggregation. Female mice of the CD1 strain were used as foster mothers. Several founder animals for each mouse line were used for establishing line stock with variable intercrosses between single founder and C57BL/6 wild-type animals. Selection of animals for analysis and breeding was random. For all animal experiments, no choice of sample size was applied. The data collection was performed according to the stage of each sample and investigators were not blinded since mouse breeding and analysis required knowledge about the genotype at hand. Routine bedding, food and water changes were performed. Mice were housed in a centrally controlled environment with a 12 h light: 12 h dark cycle, temperature of 20–22.2 C°, and humidity of 30–50%. Whole mount in situ hybridization (WISH) RNA expression in E11.5 mouse embryos from wild-type and mutants was assessed by WISH using digoxigenin (DIG)-labelled antisense riboprobes for Lbx1 , Btrc , Poll , Dpcd , Fbxw4 and Fgf8 transcribed from linearized gene-specific probes (PCR DIG Probe Synthesis Kit; Roche, Cat. #11636090910). Primers for probe generation are listed in Supplementary Table 5 . 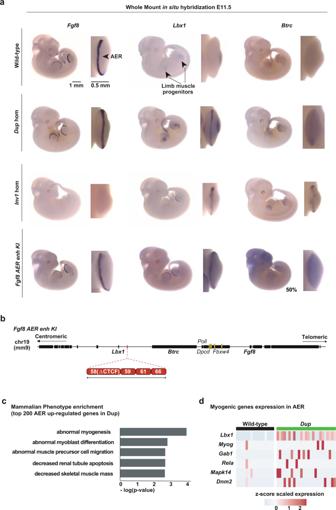Fig. 5: Ectopic interactions result inLbx1andBtrcmisexpression in the AER. aWhole-mount in situ hybridization forFgf8,Lbx1andBtrcat E11.5. Expression was checked and confirmed in at least 3 or more homozygous embryos (at leastn= 3 biological replicates).bSchematic of theLbx1/Fgf8locus for CRISPR/Cas9Fgf8 AER enhancer KIallele. Yellow ovals highlightFgf8AER enhancers.cGO analysis for the MGI Mammalian phenotype enrichment terms59using the top 200 genes that are up-regulated genes in theDupmutant compared to wild-type in the AER cells from the scRNA-seq data. The 5 most significant enriched terms are represented on a -log10 (p-value) scale.P-value was computed using a Fisher exact test.dHeatmap showing the expression of 6 genes (Lbx1, Myog, Gab1, Rela, Mapk14andDnm2) associated with the myogenic enriched terms in (c) in the AER cells. Each column represents one AER cell and the z-score scaled expression is indicated for each gene, showing a global increased expression in theDupmutant’s AER cells. Embryos were collected and fixed overnight in 4% PFA in PBS, then washed twice for 30 min in PBS with 0.1% Tween (PBST), dehydrated for 30 min each in 25%, 50% and 75% methanol in PBST and stored at −20 °C in 100% methanol. For WISH, genotyped embryos were rehydrated on ice in reverse methanol/PBST steps, washed twice in PBST, bleached in 6% H 2 O 2 in PBST for 1 h and washed in PBST. Embryos were washed in PBST and refixed for 20 min with 4% PFA in PBS, 0.2% glutaraldehyde and 0.1% Tween. After further washing steps with PBST, embryos were incubated at 68 °C in L1 buffer (50% deionized formamide, 5× SSC, 1% SDS, 0.1% Tween 20 in diethyl pyrocarbonate (DEPC), pH 4.5) for 10 min. For prehybridization, embryos were incubated for 2 h at 68 °C in hybridization buffer 1 (L1 with 0.1% tRNA and 0.05% heparin), while for subsequent probe hybridization, embryos were incubated overnight at 68 °C in hybridization buffer 2 (hybridization buffer 1 with 0.1% tRNA, 0.05% heparin and 1:500 DIG probe). The next day, unbound probes were washed away through repeated washing steps: 3 × 30 min at 68 °C with L1, L2 (50% deionized formamide, 2× SSC, pH 4.5, 0.1% Tween 20 in DEPC, pH 4.5) and L3 (2× SSC, pH 4.5, 0.1% Tween 20 in DEPC, pH 4.5). For signal detection, embryos were treated for 1 h with RNase solution (0.1 M NaCl, 0.01 M Tris, pH 7.5, 0.2% Tween 20, 100 μg ml −1 RNase A in H 2 O), followed by washing in TBST 1 (140 mM NaCl, 2.7 mM KCl, 25 mM Tris–HCl, 1% Tween 20, pH 7.5) and blocking for 2 h at room temperature in blocking solution (TBST 1 with 2% calf serum and 0.2% bovine serum albumin). Overnight incubation with Anti-Dig antibody conjugated to alkaline phosphatase (1:5,000) at 4 °C (Roche, Cat.#11093274910) was followed by 8 × 30 min washing steps at room temperature with TBST 2 (TBST with 0.1% Tween 20 and 0.05% levamisole–tetramisole) and left overnight at 4 °C. Embryos were finally stained after equilibration in AP buffer (0.02 M NaCl, 0.05 M MgCl 2 , 0.1% Tween 20, 0.1 M Tris–HCl and 0.05% levamisole–tetramisole in H 2 O) 3 × 20 min, followed by staining with BM Purple AP Substrate (Roche, Cat. #11442074001). The stained embryos were imaged using a Zeiss SteREO Discovery V12 microscope and Leica DFC420 digital camera. Skeletal preparation E18.5 fetuses were kept in H2O for 1–2 h at room temperature and heat shocked at 65 °C for 1 min. The skin was gently removed, together with the abdominal and thoracic viscera using forceps. The fetuses were then fixed in 100% ethanol overnight. Afterwards, alcian blue staining solution (150 mg l − 1 alcian blue 8GX in 80% ethanol and 20% acetic acid) was used to stain the cartilage overnight. After 24 h fetuses were rinsed and postfixed in 100% ethanol overnight, followed by 24 h incubation in 0.2% KOH in H2O for initial clearing. The next day fetuses were incubated in alizarin red (50 mg l − 1 alizarin red S in 0.2% potassium hydroxide) to stain the bones overnight. Following this, rinsing and clearing was done for several days using 0.2% KOH. The stained embryos were dissected in 25% glycerol, imaged using a Zeiss SteREO Discovery V12 microscope and Leica DFC420 digital camera, and subsequently stored in 80% glycerol. Capture Hi-C E11.5 mouse limb buds were prepared in 1x PBS and dissociated by trypsin treatment for 10 min at 37 °C, pipetting every 2 min to obtain a single-cell suspension. Trypsin was stopped by adding 5x volume of 10% FCS/PBS. The solution was then filtered through 40 μm cell strainer to remove cell debris, cells were centrifuged at 130 x g for 5 min and the pellet was then resuspended in 5 ml 10% FCS/ PBS. 5 ml of freshly prepared 4% formaldehyde in 10% FCS/PBS (final concentration 2%) were added to perform crosslinking and samples were incubated in rotation for 10 min at room temperature. The crosslinking reaction was stopped by adding 1 ml 1.425 M glycine on ice, followed by centrifugation at 240 x g and 4 °C for 8 min, pellet resuspension in 5 ml freshly prepared, cold lysis buffer (final concentration of 10 mM Tris pH 7.5, 10 mM NaCl, 5 mM MgCl2, 0.1 M EDTA, and 1 × cOmplete TM protease inhibitors (Roche, Cat. #04693132001) and incubation for at least 10 min on ice. Nuclei were pelleted by centrifugation at 425 x g at 4 °C for 5 min, washed with 1x PBS, aliquoted in 1.5 ml tubes with 2.5–5 × 10 6 nuclei each, followed by supernatant removal, snap-freezing and storage at −80 °C. Snap-frozen pellet was resuspended in 360 μl of water, mixed with 60 μl of 10x DpnII buffer (Thermo Fisher Scientific, Cat. #ER1701) and incubated for 5 min at 37 °C in a thermomixer at 900 rpm. 15 μl of 10% SDS was then added and the samples were incubated for 1 h at 37 °C and 900 rpm, with occasional pipetting to help dissolving the nuclei aggregates. Next, 150 μl of 10% Triton X-100 were added, followed by 1 h of incubation at 37 °C and 900 rpm. After adding 600 μl of 1x DpnII buffer, a 10 μl aliquot was taken as undigested control and stored at 4 °C and 400 units of restriction enzyme DpnII were added to the samples. After 4 h of digestion additional 200 units of DpnII enzyme were added and the samples were incubated overnight at 37 °C with shaking at 900 rpm. After overnight incubation, a 10 μl aliquot was taken as digested control and stored at 4 °C, while the samples were supplemented with further 200 units of DpnII enzyme for additional four hours. Meanwhile, the undigested and digested controls were tested. For this, each 10 μl aliquot was mixed with 85 μl 10 mM Tris pH 7.5 and 2 μl RNase A (10 mg/ml) and incubated for 1 h at 37 °C. Chromatin was decrosslinked by adding 5 μl proteinase K (10 mg/ ml) and incubation at 65 °C for 4 h. The DNA was then extracted by adding 100 μl phenol-chloroform. Samples were mixed by inverting the tubes and centrifuged for 10 min at 18500 x g at room temperature. The upper water phase was transferred into new 1.5 ml tubes and analysed on a 1% agarose gel. After correct validation, restriction enzyme in the original samples still under digestion was heat-inactivated at 65 °C for 20 min. The samples were transferred to 50 ml Falcon tubes and 700 μl 10x ligation buffer (Thermo Fisher Scientific, Cat. #EL0021) were added. The volume was filled up to 7 ml with water and 50 units of T4 DNA ligase (Thermo Fisher Scientific, Cat. #EL0021) were added. The ligation mix was incubated overnight at 4 °C in rotation. The next day, a 100 μl aliquot of religated DNA was collected and analysed on an agarose gel as described above. Upon successful ligation, samples were de-crosslinked by adding 30 μl of proteinase K (10 mg/ml) and incubating overnight at 65 °C. Then, 30 μl RNase A (10 mg/ml) were added and the samples were incubated for 45 min at 37 °C. The DNA was then extracted by adding 7 ml phenol-chloroform. The solution was mixed by inverting the tube and the water phase was separated by centrifugation at 1500 x g for 15 min at room temperature. DNA was precipitated by adding the following reagents to the water phase: 7 ml water, 1.5 ml 2 M NaAc pH 5.6, 140 μg glycogen, 35 ml 100 % ethanol. The solution was mixed and placed at −80 °C overnight or until the samples were completely frozen. The sample was then thawed and centrifuged for 20 min at 8350 g and 4 °C. DNA pellet was washed with 30 ml cold 70% ethanol and centrifuged 15 min at 3300 g at 4 °C. Dried pellet was dissolved in 150 μl 10 mM Tris pH 7.5 at 37 °C. The final 3 C library was checked on 1% agarose gel and subsequently used for capture Hi-C preparation. 3 C libraries were sheared using a Covaris sonicator (duty cycle: 10%; intensity: 5; cycles per burst: 200; time: 6 cycles of 60 s each; set mode: frequency sweeping; temperature: 4–7 °C). Adaptors were added to the sheared DNA and amplified according to Agilent instructions for Illumina sequencing. The library was hybridized to the custom-designed SureSelect beads and indexed for sequencing following Agilent instructions. SureSelect enrichment probes were designed over the genomic interval chr19:44,440,000-46,400,000 (mm9) using the online tool of Agilent: SureDesign ( https://earray.chem.agilent.com/suredesign/ ). Probes were covering the entire genomic region and were not designed specifically in proximity of DpnII sites. All samples (3 biological replicates per experiment plus one technical, except for Inv1 het where no technical replicate was produced, and for Dup het where only one biological replicate was used) were then sequenced with the Hiseq4000 or Novaseq6000 Illumina technology according to the standard protocols and with around 400 million 50 bp, 75 bp (Hiseq4000) or 100 bp (Novaseq6000) paired-end reads per sample. Capture Hi-C data processing In a pre-processing step, the reads in fastq files were trimmed to 50 bp, if necessary, to obtain the same initial read length for all samples. Afterwards, mapping, filtering and deduplication of paired-end sequencing data was performed using the HiCUP pipeline v0.8.1 [46] (no size selection, Nofill: 1, Format: Sanger). The pipeline was set up with Bowtie2 v2.4.2 [47] for mapping short reads to reference genome mm9. For merging biological replicates, the final bam files produced by the HiCUP pipeline were joined. 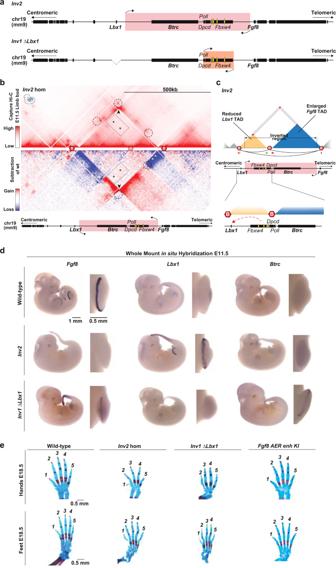Fig. 6: Misexpression of bothLbx1andBtrcis required to develop a SHFM phenotype. aSchematics of theLbx1/Fgf8locus for CRISPR/Cas9Inv2andInv1 ∆Lbx1alleles. Yellow ovals highlightFgf8AER enhancers.bcHi-C (data are shown as merged signal ofn= 3 biological and 1 technical replicates) of homozygousInv2from E11.5 mouse limb buds. The subtraction map between wild-type andInv2interactions is shown in mirror view. Dashed circles indicate the position of the original wild-type interactions between boundaries, two of them lost upon reshuffling of the boundary betweenLbx1andFgf8TADs as a consequence of this inversion. The boundary involved in the inversion is shown as blurry. Black arrowhead highlights the bow tie configuration representative of the inverted regions. The rectangular dashed area highlighted by black asterisks show ectopic interactions compared to wild-type between theFgf8AER enhancers region and the one containing now onlyLbx1and not anymoreBtrc. White asterisks point out the loss of interactions betweenFgf8and its AER enhancers.cSchematic ofInv2configuration. Upon this inversion, theFgf8AER enhancers are repositioned within a smallerLbx1TAD, whereas theFgf8TAD is increased in size due to the inversion of the boundary and contains nowBtrc, isolated from theFgf8AER enhancers. Below is a zoom-in of the locus highlighting the potential ectopic interactions (red dashed arrow) involving theFgf8AER enhancers now repositioned within theLbx1TAD.dWhole-mount in situ hybridization forFgf8,Lbx1andBtrcat E11.5. Expression was checked and confirmed in at least 3 or more homozygous embryos (at leastn= 3 biological replicates).eSkeletal analysis of E18.5 limbs stained with alcian blue (cartilage) and alizarin red (bone). Hands and feet from wild-type,Inv2, Inv1 ∆Lbx1andFgf8 AER enhancer KIE18.5 embryos. At leastn= 3 biological replicates. 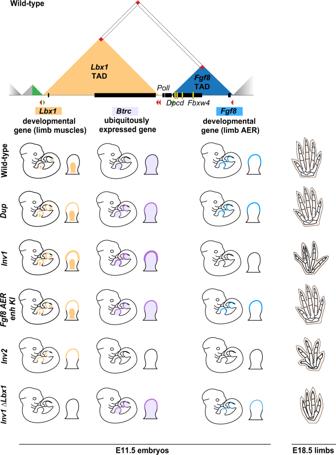Fig. 7: Combinatorial effects on gene expression at theLbx1/Fgf8locus leads to SHFM3 digit fusion phenotype. Schematic overview of theLbx1-Fgf8TADs (top) andLbx1,BtrcandFgf8expression in the developing limb at E11.5 and skeletal phenotype at E18.5 among the different structural rearrangements (bottom). Yellow and violet patterns represent endogenous expression in the limb bud and misexpression in the AER ofLbx1andBtrc, respectively. Turquoise pattern highlightsFgf8expression in the AER. Ectopic expression of bothLbx1andBtrcin the AER is observed for theDup,Inv1andFgf8AER enhancer KI (Fgf8 AER enh KI) mutant embryos at E11.5. However, only theInv1mutants, for which the level ofLbx1andBtrcexpression in the AER is higher andFgf8expression is missing, show a digit fusion phenotype at E18.5, reminiscent of human SHFM. Ectopic expression of eitherLbx1alone (Inv2mutant) orBtrcalone (Inv1 ΔLbx1mutant) together with complete (Inv2) or partial (Inv1 ΔLbx1) loss ofFgf8AER expression is not enough to lead to the digit fusion SHFM-like phenotype but only results in anFgf8-KO limb phenotype. Juicer tools v1.19.02 [48] d was used to generate binned and KR normalized [49] , [50] contact maps from valid and deduplicated read pairs. For the generation of cHi-C maps, only read-pairs referring to the region of interest (chr19:44,440,001-46,400,000) and with MAPQ ≥ 30 were considered. We used cHi-C maps with 5 kb bin size. For the sample with a duplication it is noted, that the matrix balancing of the KR normalization affects the signal in the duplicated region, because it scales down the signal intensities in this region to fit to the other regions of the cHi-C map. In order to consider the duplicated region explicitly, we created for the Dup mutant sample an additional version of the cHi-C map by applying LOIC normalization [51] (python package iced v.0.5.10 [52] ) to raw count map, which has the aim to retain the effects of the increased copy number. For the LOIC normalization the copy number was set to 4 for all bins overlapping the duplication, and to 2 for the other bins. For five matrix rows/columns with low coverage, the count values were removed prior to LOIC-normalization. Subtraction maps were computed from KR-normalized cHi-C maps, which were normalized in a pairwise manner before subtraction as follows. To account for differences between two maps in their distance-dependent signal decay, the maps were scaled jointly across their sub-diagonals. Therefore, the values of each sub-diagonal of one map were divided by the sum of this sub-diagonal and multiplied by the average of these sums from both maps. Afterwards, the maps were scaled by 10 6 /total sum. For the computation of scaling factors, the duplicated as well as the inverted regions were excluded in both maps. cHi-C maps were visualized as heatmaps with linear scale, with very high values being truncated to improve visualization. Virtual 4C Virtual 4C-like interaction profiles were generated for individual viewpoints from the same bam files also used for the cHi-C maps. Paired-end reads with MAPQ ≥ 30 were considered in a profile, when one read mapped to the defined viewpoint region and the other one outside of it. Contacts of a viewpoint region were counted per restriction fragment. The count profile was binned to a 1 kb grid. In case a fragment overlapped more than one bin, the counts were distributed proportionally. Afterwards, the binned profile was smoothed by averaging within a sliding window of 5 kb size and scaled by 10 3 /sum of counts within the enriched region. The viewpoint region itself and a margin ±5 kb around it were excluded from the computation of the scaling factor. Interaction profiles were generated with custom Java code using v2.12.0 ( https://samtools.github.io/htsjdk/ ). RNA expression analysis E11.5 limb buds were microdissected from wild-type and mutant embryos (at least n =  3) and immediately frozen in liquid nitrogen. Total RNA was isolated using the RNeasy Mini Kit (Qiagen, Cat. #74004). For RNA-sequencing, samples were poly-A enriched and sequenced with the Novaseq6000 Illumina technology according to the standard protocols and with around 100 million 100 bp paired-end reads per sample. For RT-qPCR, cDNA was generated using 1 ug of extracted RNA and reverse transcribed using Superscript III (Life Technologies, Cat. # 18080093) with oligo(dT) 25 as template primers. 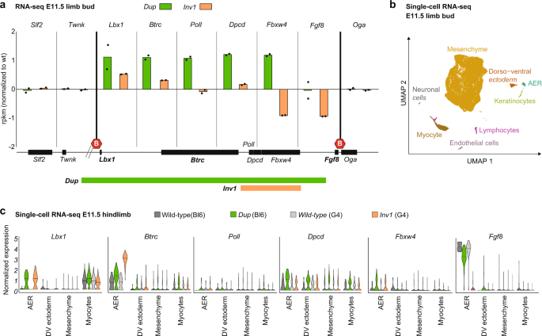RT-qPCR was performed using the Biozym Blue S’Green qPCR Mix Separate ROX (Biozym, Cat. # 331416 S). Relative expression levels were normalized to the geometric mean of the Ct for housekeeping genes Rrm2 and Rplp0 , with the ΔΔCt method and data were shown as normalized to WT values. Fig. 4:DupandInv1chromatin rearrangements have an impact on gene expression. aBar plot representing the rpkm value normalized to wild-type for genes in theLbx1andFgf8TADs and flanking genes (Slf2andTwnk(centromeric),Oga(telomeric)) from RNA-seq data of homozygousDupandInv1E11.5 limb buds.n= 2 biological replicates per condition. Schematic of the locus shows the position of the genes, the TAD boundaries (red hexagons) and the parts included in the Dup and the Inv1 mutants. Wild-typeDupandInv1samples are shown in black, green and orange, respectively.bUniform manifold approximation and projection (UMAP) showing 8 cell clusters identified via scRNA-seq of E11.5 mouse limbs from wild-type,DupandInv1mutants (n= 1).cViolin plot representing the normalized expression of the 6 genes at the locus in AER, dorso-ventral (DV) ectoderm, mesenchyme and myocytes from E11.5 hindlimbs. TheDupmutant (green) was generated in a C57Bl6 background and thus compared to a C57Bl6 wild-type sample (dark grey) whereas theInv1mutant (orange) was generated in a G4 (129sv x C57Bl6) and compared to a G4 wild-type sample (light grey). Primers used are listed in Supplementary Table 4 . RNA-seq data processing Reads were mapped to the mouse reference genome (mm9) using the STAR mapper [53] (splice junctions based on RefSeq; options: –alignIntronMin 20–alignIntronMax 500000–outFilterMultimapNmax 5–outFilterMismatchNmax 10–outFilterMismatchNoverLmax 0.1). Reads per gene were counted as described previously [3] , and used for differential expression analysis with the DEseq2 package [54] . scRNA-seq scRNA-seq experiments were performed in single replicates that were jointly processed to avoid batch effects. E11.5 limb buds of wild-type, Dup and Inv1 embryos were microdissected in 1xPBS at room temperature. A single-cell suspension was obtained by incubating the tissue for 10 min at 37 °C in 200 μl Gibco trypsin-EDTA 0.05% (Thermo Fisher Scientific, Cat. #25300054) supplemented with 20 μl 5% BSA. Trypsinization was then stopped by adding 400 μl of 5% BSA. Cells were then resuspended by pipetting, filtered using a 0.40 μm cell, washed once with 0.04% BSA, centrifuged for 5 min at 150 x g , then resuspended in 0.04% BSA. The cell concentration was determined using an automated cell counter (Bio-Rad) and cells were subjected to scRNA-seq (10x Genomics, Chromium Single Cell 3′ v2; one reaction per time point and per strain has been used) aiming for a target cell recovery of up to 10,000 sequenced cells per sequencing library (time point and strain). Single-cell libraries were generated according to the 10x Genomics instructions with the following conditions: 8 PCR cycles were run during cDNA amplification and 12 PCR cycles were run during library generation and sample indexing to increase library complexity. Libraries were sequenced with a minimum of 230 million 75 bp paired-end reads according to standard protocols. scRNA-seq data processing The Cell Ranger pipeline v.3 (10x Genomics lnc.) was used for each scRNA-seq sample in order to de-multiplex the raw base call files, to generate the fastq files, and to perform the alignment against a custom mouse reference genome mm9 to create the unique molecular identifier (UMI) count matrix. Only cells with more than 2000 detected genes and less than 10% of mitochondrial UMI counts were considered for further analysis. In addition, Scrublet [55] was used to identify potential doublets in our dataset. Cells with a Scrublet score higher than 0.2 were filtered out. Each sample was normalized independently using the SCT method [56] implemented in Seurat [57] R package and then, these were integrated using the Seurat3 IntegrateData CCA-based (canonical correlation analysis) approach considering the top 2,000 most variable genes. The first 20 principal components of this joint dataset were calculated and used for UMAP projection and reconstruction of the cell-cell similarity graph. To delimitate the major limb bud cell types, we used the Louvain algorithm implemented in the Seurat3 function FindClusters and the expression of well-known marker genes for the limb-comprising cell types. For the AER cluster, we used the marker genes Fgf8 and En1 . Differential gene expression between the wild-type (Bl6) vs Dup and wild-type (G4) vs Inv1 hindlimb cells was estimated by modelling the gene expression as a function of the genotype across cells. This analysis was done from a new embedding of the samples separately: on one hand wild-type (Bl6) and Dup , on the other hand wild-type (G4) and Inv1 . We fitted a quasi-Poisson distribution to calculate the effect of the Dup or the Inv1 genotype on the gene expression distribution of each gene using the monocle3 strategy [58] . We tested that such effect was not equal to 0. We use this condition association effect to rank the genes and identified the pathways associated with the top 200 genes using the Enrichr tool from the Maayan lab [59] . Finally, we confirmed that the top perturbed genes associated to the muscle pathways are more frequently expressed in the Dup AER cells. 4C-seq For 4C-seq libraries, 5 × 10 6 –10 7 cells were used. The fixation and lysis were performed as described in the Capture Hi-C section. After the first digestion with DpnII, sticky ends were religated in a 50 ml falcon tube (700 μl 10X ligation buffer, 7 ml H2O, 50 U T4 DNA ligase; overnight at 16 °C) and DNA de-cross linked and cleaned as described in the Capture Hi-C section. Next, a second digestion (150 μl sample, 50 μl 10× Csp6I buffer, 60 U Csp6I (Thermo, Cat. # FD0214) 295 μl H2O; overnight at 37 °C) and another re-ligation were performed. For all viewpoints, DNA was purified using a PCR clean up Kit (Qiagen, Cat. #28104) and 1.6 μg DNA was amplified by PCR ( LBX1 Viewpoint: read-primer 5′-TCTATATGCTACCATGATC-3′, secondary-primer 5′-GATGAACTGGAATACCCA-3′; FGF8 Viewpoint: read-primer 5′-AGGGTGCGTTCCAAGATC-3′, secondary-primer 5′-GGTGGCCTGGATGGAAGT-3′; BTRC Viewpoint: read-primer 5′-CAACGCAGCGCCCGGATC-3′, secondary-primer 5′-CTGGGAATGAGGACCTAGGGC-3′). For the library reaction, primers were modified with TruSeq adapters: Adapter1 5′-CTACACGACGCTCTTCCGATCT-3′ and Adapter2 5′-CAGAC GTGTGCTCTTCCGATCT-3′. Between 50 and 200 ng were used as input of a single 4C PCR reaction depending on the complexity. The reaction was performed in a 50 μl volume using the Expand Long Template System (Roche, Cat. # 11681834001) and 29 reaction cycles. After the PCR all reactions were combined and the DNA purified with a PCR clean up Kit. All samples were then sequenced with the Novaseq6000 Illumina technology according to the standard protocols and with around 5 million 100 bp single-end reads per sample. 4C-seq data processing Sequencing reads were mapped, normalized and smoothed with pipe4C [60] using the reference genome GRCh37 and default settings. All viewpoints were performed in replicates and as quality measure >70% of reads were mapped within a size range of 1 Mb and >80% within 100 kb around the viewpoint. Human material Skin biopsies were collected from SHFM3 patients and controls by standard procedures. Fibroblasts were cultured in DMEM supplemented with 10% fetal calf serum (Gibco, Cat. #A4766801), 1% L-glutamine (Lonza, Cat. #BE17-650E) and 1% penicillin/streptomycin (Fisher, Cat. #BP295950). Reporting summary Further information on research design is available in the Nature Portfolio Reporting Summary linked to this article.